Unsupported boron–carbon σ-coordination to platinum as an isolable snapshot of σ-bond activation σ-Complexes of transition metals—key intermediates in metal-mediated bond activation and homogeneous catalysis—have traditionally been isolable only when chelating or when one of the participating atoms is hydrogen. Here, by treating the Lewis-basic transition metal complex [Pt(PEt 3 ) 4 ] with an electron-poor borirene, we isolate a complex with an unsupported borirene ligand bound, not through the unsaturated C=C bond, but exclusively via a B–C single bond. Using NMR spectroscopy, X-ray crystallography and density functional theory calculations, we show, herein, that coordination of the borirene ligand is based on electron donation from the B–C σ bond to the metal, aided by a strong Pt-to-B dative interaction. The complex is the first isolable non-agostic σ-complex featuring two p -block elements and has broad implications as a model for the metal-mediated activation of strong p -block- p -block σ-bonds. Transition metals are indispensable in catalysis because of their ability to break and form σ-bonds between main-group elements. A seemingly simple prerequisite for metal activation of element–element (E-E) σ bonds is that the bond must come near the metal centre—requiring some energetic payoff for the steric inconvenience of bringing the fragments together. This payoff is generally provided by electron donation from the filled E-E σ orbital to the metal (interaction I , Fig. 1a ), forming a usually transient state known as a σ-complex [1] , [2] . Few σ-complexes have garnered as much attention as the σ-alkanes, putative intermediates in the catalytic C–H functionalization of alkanes, the pursuit of which has occupied researchers worldwide for decades [3] , [4] , [5] , [6] , [7] . A number of σ-alkane complexes have been characterized at low temperature by NMR, but the only structurally characterized examples are topics of debate [8] , [9] . Isolable σ-complexes range from complexes with weak agostic (that is, supported by a stronger secondary point of ligation) C–H [10] , [11] , C–C [12] , [13] and Si–Si [14] , [15] ligation to strong, unsupported σ-dihydrogen [1] , [2] and σ-borane complexes [16] , [17] , [18] , [19] , [20] , [21] , [22] , [23] , whose stability (significantly enhanced in the latter by retrodonation interaction III , Fig. 1a ) has led to advances in our understanding of catalytic hydrogenation, hydroboration [24] , [25] , [26] , and reversible hydrogen storage by amine-boranes [27] , [28] , [29] . 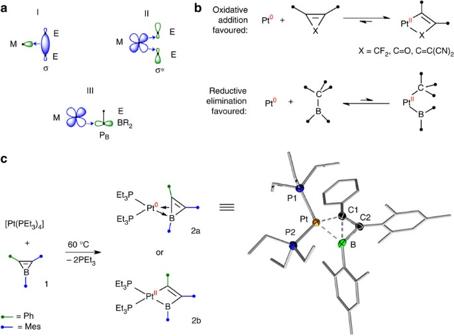Figure 1: Overview of relevant bonding and synthetic aspects. (a) Known bonding modes of relevance to σ-complexes. For E=H, a singlesorbital centred at H participates instead of those pictured. (b) Documented preferences of platinum systems with certain ligand fragments. (c) Synthesis and solid-state molecular structure of complex2reported herein. Mes, mesityl. Thermal ellipsoids depicted at the 50% probability level. For clarity, hydrogen atoms have been removed and thermal ellipsoids are not shown for the ligand backbones. Selected bond lengths (Å) and angles (°) for2: Pt-B 2.121(7), Pt-C1 2.067(7), B–C1 1.89(1), B–C2 1.54(1), C1-C2 1.38(1), Pt1-P1 2.341(2), Pt-P2 2.273(2); C1-C2-B1 80.7(5), P2-Pt-P1 104.03(7). 'Butterfly' angle between Pt-B–C1 and B–C1-C2 planes: 137.35°. Figure 1: Overview of relevant bonding and synthetic aspects. ( a ) Known bonding modes of relevance to σ-complexes. For E=H, a single s orbital centred at H participates instead of those pictured. ( b ) Documented preferences of platinum systems with certain ligand fragments. ( c ) Synthesis and solid-state molecular structure of complex 2 reported herein. Mes, mesityl. Thermal ellipsoids depicted at the 50% probability level. For clarity, hydrogen atoms have been removed and thermal ellipsoids are not shown for the ligand backbones. Selected bond lengths (Å) and angles (°) for 2 : Pt-B 2.121(7), Pt-C1 2.067(7), B–C1 1.89(1), B–C2 1.54(1), C1-C2 1.38(1), Pt1-P1 2.341(2), Pt-P2 2.273(2); C1-C2-B1 80.7(5), P2-Pt-P1 104.03(7). 'Butterfly' angle between Pt-B–C1 and B–C1-C2 planes: 137.35°. Full size image The metal-mediated stoichiometric and catalytic borylation of alkanes and arenes had far-reaching implications for synthetic chemistry [30] , [31] , [32] , [33] , [34] , [35] , [36] . The final steps of this reaction include B–C bond formation on the metal centre and ejection of the formed organoborane molecule. Lin calculated minima for this step, in which formed alkylboranes bind weakly through C–H σ-coordination to the metal before elimination, while arylboranes bind through B–C 1 =C 2 aryl carbon atoms [37] . In contrast, Hartwig, Webster and Harris computationally implicated a B–C σ-complex as the final intermediate in metal-mediated alkane borylation—suggesting the feasibility of a new type of σ-complex of relevance to both the formation and cleavage of B–C bonds [38] . Carbon–boron single bonds (358 kJmol −1 ) are among the strongest single bonds involving carbon, stronger than C–C bonds (346 kJmol −1 ) and approaching C–H bonds (411 kJmol −1 ). Isolated reports of oxidative addition of B–C bonds to transition metals exist [39] , [40] , making activation of this bond an intriguing target. Facile oxidative addition of cyclic C–C single bonds to Pt 0 has been documented with cyclopropenones [41] , methylenecyclopropenes [42] and tetrafluorocyclopropene [43] ( Fig. 1b ), while examples of B–B oxidative addition are numerous [44] . Thus, we questioned whether boron analogues borirenes ( cyclo -BC 2 R 3 ) might be similarly susceptible to B–C bond rupture. This was by no means certain, as platinum cis -(σ-organyl)(boryl) complexes are known to be extremely unstable, preferring reductive elimination and formation of the strong B–C bond, an effect put to use in transition metal-catalysed diboration reactions ( Fig. 1b ) [45] . We have had an interest in borirenes for some time [46] , [47] , [48] , however, in our hands, B -aminoborirenes have so far been inactive towards low-valent transition metals. The only known coordination chemistry of borirenes is the step-wise assembly of a η 3 :μ 3 -(2-methylborirene) unit on a Fe 3 (CO) 9 cluster core by Fehlner, suggesting a possible preference for π-coordination of borirenes to transition metals [49] . To best promote the coordination chemistry of such electron-poor borirenes, we turned first to strongly Lewis basic fragments of zero-valent platinum. Here we present the synthesis of a platinum σ-complex in which an unsupported borirene ligand is bound solely through a boron–carbon single bond, the apparent result of an incomplete B–C bond oxidative addition reaction. Synthesis and characterization of 2 To induce a reaction with a Pt 0 fragment, 1,2-dimesityl-3-phenylborirene ( 1 ), a borirene lacking stabilizing π-donor groups, was treated with in-situ generated [Pt(PEt 3 ) 2 ]. The pale yellow solid 2 was isolated and confirmed to be a 1:1 coordination complex of the borirene and the [Pt(PEt 3 ) 2 ] fragment. The borirene ligand seems strongly bound to Pt; however it can be displaced by diphenylacetylene yielding [(Et 3 P) 2 Pt( η 2 -PhCCPh)] and free borirene. This observation suggested that the structure of 2 might resemble a σ-bond complex, which are often easily displaced by superior donor ligands. The 31 P NMR spectrum of 2 showed that the two phosphine ligands were mutually cis coordinated and that the borirene was bound in an unsymmetrical fashion—, that is, not a simple η 2 -olefin complex with the borirene C=C bond, nor a symmetrical η 3 -borirene complex similar to that of Fehlner [49] . The 13 C{ 1 H} NMR spectrum of 2 ( Supplementary Figs S1 and S2 ) shows a downfield movement of the Pt-bound carbon nucleus ( 1 : 171; 2 : 189 p.p.m. ), whereas the remaining borirene carbon remains practically unchanged ( 1 : 167; 2 : 166 p.p.m. ), suggesting that the environment of only one of the two nuclei has been altered. Both borirene carbon nuclei are broadened owing to coupling to 11 B, and no coupling could be observed for the Pt-bound carbon signal. A partially resolved 13 C- 11 B coupling of ca. 80 Hz can be observed for the remaining borirene carbon atom, suggesting a stronger connection to the boron atom than that bound to Pt. The 11 B NMR signal of 2 is also shifted downfield by a small amount ( 1 : 32.8; 2 : 39.6 p.p.m.) on complexation. X-ray crystallographic analysis ( Fig. 1c ; Supplementary Fig. S3 ; see the Supplementary Methods section for crystal data) showed the Pt centre to be bound to the B and one C atom of the borirene, and that the Pt-B–C and B–C–C planes of 2 form a butterfly structure (angle between planes: 137.35°), almost exactly mid-way between that expected for a purely π -bound complex (ca. 90°) and the coplanar structure observed by Hughes in the tetrafluorometallacyclobutene complex cis -[(Ph 3 P) 2 Pt(κ 2 -C 3 F 4 )] (177.68°) [43] . This butterfly structure provides a clear indication that 2 does not fit a 'metallacyclobutene' description, suggesting that, at most, only partial oxidative addition of the B–C bond has occurred. The angles at the non-metal-bound carbon atom of known Pt II metallacyclobutenes (100°, 101° and 104.7(7)°) [41] , [42] , [43] are diagnostic for a 'complete addition' description, while the analogous angle in 2 (80.7(5)°) suggests that the BC 2 ring is significantly more intact. Calculations by Sakaki show that the B–C distances in the transition state structures of Pt-mediated activation of the B–C bond of H 3 C-B(OH) 2 are in the range 1.687–1.756 Å, both considerably shorter than the B–C distance in 2 (1.89(1) Å), but longer than the B–C distance in the free borirene (1.459(4) Å; Supplementary Fig. S4 ) [50] . Moreover, Frenking's calculation of borirene B–C bond breakage involved a B–C transition state distance of 1.525 Å (ref. 51 ). Maron, Bouhadir and Bourissou have reported agostic B( sp 2 )-C( sp 2 ) bonds side-on bound to Cu I ; however, these bonds show no significant elongation (1.566(3) Å) and appear very weakly bound to the metal [52] . These three studies suggest that the relatively long B–C distance of 2 can no longer be classified as a full single bond. On the other hand, this B–C distance fits a broken-bond description very poorly. Sakaki predicts B–C distances of 2.336-2.611 Å (149-166% of the sum of the covalent radii, Σ covrad ) in B–C bond oxidative addition products cis -[(R 3 P) 2 Pt{B(OH) 2 }(CH 3 )] (R 3 =H 3 , H 2 Me, H 2 Et). 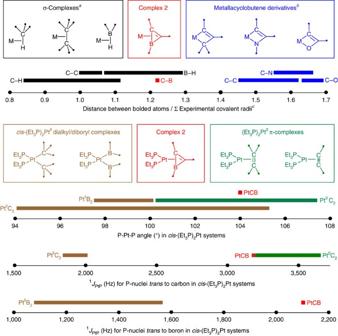Figure 2: Analysis of various metrics related to complex 2 derived from X-ray crystallography and31P NMR spectroscopy. aC–H distances in agostic complexes derived from neutron diffraction.bOnly metallacyclobutene derivatives with two definitive covalent metal-element bonds were considered, complexes with dative M←N(R)2C=C or M←O(R)C=C interactions were ignored.cExperimental covalent radii were derived from a published survey of the Cambridge Crystallographic Database54. Figure 2 shows that analogous distances in metallacyclobutene derivatives in which BR is replaced with CR 2 , NR or O (145–169% of Σ covrad ) are all significantly longer than that of 2 (121% of Σ covrad )—this includes highly comparable platinacyclobutene structures [41] , [42] , [43] . The Pt-C distance in 2 is within the range found in classical óσ-vinyl complexes, whereas the Pt-B distance is slightly longer than those found in Pt-boryl complexes, although a part of this lengthening could stem from the bulky mesityl group at boron [53] . Nevertheless, a description involving complete Pt-insertion into the borirene fragment is incompatible with the observation of such a short B–C distance. Figure 2 shows two additional metrics (P-Pt-P angle and 1 J PtP values) that compare 2 with related cis -[(Et 3 P) 2 PtL n ] complexes containing both Pt 0 and Pt II centres, both of which strongly support the description of the complex as a Pt 0 complex. These metrics indicate that the broken-bond metallacyclobutene structure corresponding to structure 2b ( Fig. 1 ) is not an accurate model for 2 , whereas the B–C óσ-borane structure with a strong Pt-to-B dative bond 2a fits much better. As unsupported B–C σó-complexes like 2a have no precedent in the literature, empirical evaluation of the bonding description has limited utility; thus, we turned to computation to gain further insight. Figure 2: Analysis of various metrics related to complex 2 derived from X-ray crystallography and 31 P NMR spectroscopy. a C–H distances in agostic complexes derived from neutron diffraction. b Only metallacyclobutene derivatives with two definitive covalent metal-element bonds were considered, complexes with dative M←N(R) 2 C=C or M←O(R)C=C interactions were ignored. c Experimental covalent radii were derived from a published survey of the Cambridge Crystallographic Database [54] . Full size image Computational analysis of the bonding of 2 Kohn-Sham Density Functional Theory calculations (see Supplementary Methods for more details on the computational methodology) at the B3LYP/Def2-SVP level were undertaken of [Pt(PEt 3 ) 2 ] ( Supplementary Fig. S5 ), 1 ( Supplementary Fig. S5 ) and 2 ( Supplementary Fig. S6 ) without simplification of groups. The obtained geometry of 2 ( Supplementary Fig. S5 ) was used for subsequent calculation of a methylenecyclopropene analogue in which the 'BMes' fragment is replaced with 'C=CH 2 ', cis -[(Et 3 P) 2 Pt{κ 2 -H 2 C=CC(Mes)=C(Ph)}] ( 3 ). Calculations reproduced the experimental geometry of 2 well ( Fig. 3 ; Supplementary Table S1 ), with an elongated B–C bond (calcd: 1.861 Å; X-ray: 1.89(1) Å) and butterfly structure (angle between planes, calcd: 136.54°; X-ray, 137.35°). Initial enforcement of a complex containing an η 2 - C,C -borirene ligand led to a π -olefin structure 2′ ( Supplementary Fig. S7 ), found to be 5.5 kcal mol −1 less stable than 2 . The calculated methylenecyclopropene model 3 matched the literature structures of platinacyclobutene complexes with a completely broken C–C bond (calcd: 2.239 Å; literature: 2.15–2.24 Å) and coplanar arrangement of the Pt-C–C and C–C–C planes (angle between planes: 176.9) [41] , [42] , [43] . The difference between the calculated geometries of 2 and 3 are also apparent from the Wiberg bond indices of the bonds between the cyclic fragment and the Pt, with the B–C bond of 2 (WBI: 0.54) being much more complete than the C–C bond of 3 (WBI: 0.10). This incomplete cleavage of the B–C bond is also reflected by a reduction in the calculated B–C spin–spin coupling constant of the Pt-bound atoms in 2 ( J BC =−15.8 Hz) compared with the free borirene 1 ( J BC =47.0 Hz). The Pt–C interaction in 2 (WBI: 0.39) is also less intense than the corresponding bond of 3 (WBI: 0.51), indicating a more complete bond activation in 3 . From analysis of the natural bonding orbitals of relevance to the Pt–B–C core of 2 , we see in Fig. 3 that the major interactions are donation from the B–C óσ-bond to the Pt ( c . f . interaction I , Fig. 1 ), along with a strong Pt-to-B dative interaction ( c . f . interaction III , Fig. 1 ). This is supported by the observation of a much larger influx of electron density to the boron atom of 2 on complexation (partial charges, free, +0.80; bound, +0.46; net change, 0.34 e) than to C1 (partial charges, free, −0.12; bound, −0.25; net change, 0.13 e; see Supplementary Fig. S8 ). We see little computational evidence for retrodonation from Pt into the B–C óσ*orbital (that is, interaction II , Fig. 1 ), which may explain the incomplete activation of the B–C bond (for additional views, see Supplementary Figs S9–S11 ; Supplementary Table S2 contains the natural bonding orbitals (NBOs) that constitute the HOMO and HOMO-1 orbitals). 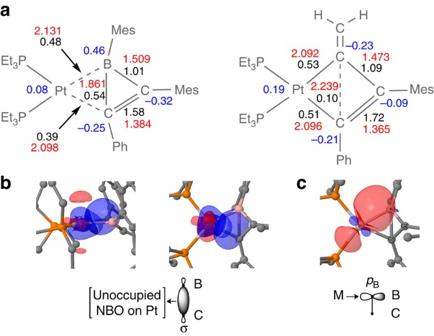Figure 3: Results of DFT calculations on complexes2and3. (a) calculated bond lengths (in red, Å), Wiberg bond indices (in black) and natural charges (in blue). Mes, mesityl. (b) Two views of the NBOs that comprise the donation from the B–C σ-bond to the metal. (c) View of the NBO corresponding to the metal-to-boron donation. Figure 3: Results of DFT calculations on complexes 2 and 3 . ( a ) calculated bond lengths (in red, Å), Wiberg bond indices (in black) and natural charges (in blue). Mes, mesityl. ( b ) Two views of the NBOs that comprise the donation from the B–C σ-bond to the metal. ( c ) View of the NBO corresponding to the metal-to-boron donation. Full size image Electrochemical properties of 2 To establish a better oxidation state description of the Pt center, we performed electrochemical measurements on 2 , finding a distinctive oxidation wave in the cyclic voltammogram at 0.03 V vs ferrocene ( Fig. 4 ). The cyclic voltammogram of a set of Pt 0 complexes measured under identical conditions show similar waves in the range −0.04 to 0.07 V, most likely representing the Pt 0 -to-Pt II oxidation process. Conversely, the Pt II complex trans -[PtCl 2 {P(CH 2 C 6 H 11 ) 3 } 2 ] showed no oxidation wave within the electrochemical window (up to +0.5 V vs ferrocene). These results lend support to the assignment of 2 as a Pt 0 species. 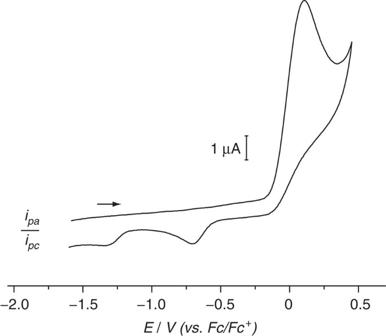Figure 4: Cyclic voltammogram of complex 2. The cyclic voltammetry was performed on a 0.1-MnBu4NPF6/THF solution at a voltage sweep rate of 0.2 V s−1. The potential scale is referenced to the ferrocene/ferrocenium couple. Figure 4: Cyclic voltammogram of complex 2. The cyclic voltammetry was performed on a 0.1-M n Bu 4 NPF 6 /THF solution at a voltage sweep rate of 0.2 V s −1 . The potential scale is referenced to the ferrocene/ferrocenium couple. Full size image The overall picture presented by experiment and computation for complex 2 is as follows: X-ray crystallography, NMR spectroscopy, cyclic voltammetry and DFT calculations all indicate that the description of complex 2 as a Pt II , B–C activated metallacyclobutene ( 2b , Fig. 1c ) is false. Calculations on model complex 3 confirm the massive chasm between the structure of metallacyclobutenes and 2 . Structure 2a ( Fig. 1c ), that is, a donation from the B–C σ-bond to Pt 0 supported by Pt-to-B dative bonding, is much more representative. Presumably, this Pt-to-B dative bond allows the ligand to bind strongly enough that no secondary ligation site is necessary. DFT calculations suggest that the Pt→ p B donation ( III , Fig. 1a ) predominates over Pt→σ* BC donation ( II ). The suppression of the latter may account for the reluctance of complex 2 to fully activate the B–C bond and adopt a planar metallabutene structure akin to 3 . General synthetic procedures All manipulations were performed under an inert atmosphere of dry argon using either standard Schlenk-line or glovebox techniques. Deuterated solvents were dried over molecular sieves and degassed by three freeze-pump-thaw cycles before use. All other solvents were distilled from appropriate drying agents [55] . Solvents were stored under argon over activated molecular sieves. Photolytic experiments were performed in quartz Schlenk flasks. The light source was a LOT-Oriel photolysis apparatus with a 500 W Hg/Xe arc lamp equipped with infrared filters, irradiating at 210–600 nm. NMR spectra of isolated compounds were acquired on a Bruker Avance 500 NMR spectrometer. Routine NMR measurements were performed on a Bruker Avance 400 NMR spectrometer. Chemical shifts (δ) are given in p.p.m. 1 H and 13 C{ 1 H} NMR spectra were referenced to external tetramethylsilane via the residual protio solvent (1 H) or the solvent itself ( 13 C). 11 B{ 1 H} NMR spectra were referenced to external BF 3 ·OEt 2 , 31 P{ 1 H} NMR spectra to 85% H 3 PO 4 and 195 Pt{ 1 H} NMR to 1.2 M Na 2 [PtCl 6 ] in D 2 O. Infrared data were acquired on a JASCO FT/IR-6200typeA apparatus. Melting points were measured with a Mettler Toledo DSC 823. Microanalyses were performed on an Elementar vario MICRO cube elemental analyser. Cq refers to quaternary carbon nuclei. Preparation of 1,2-dimesitylene-3-phenylborirene 1 The borirene was synthesized by a modified protocol of Eisch [56] . In a quartz Schlenk flask 1.00 g (2.85 mmol) of dimesitylborylphenylacetylene was dissolved in 20 ml hexane. The reaction mixture was photolysed for 24 h. NMR indicated total conversion. The solution was stored for 2 days at −60 °C. The borirene was isolated as a white solid (0.89 g, 2.54 mmol, 89%). For further purification, the borirene can be sublimed at 100°C and 2·10 −6 bar. Crystals suitable for X-ray analysis were obtained after storing a hexane solution of the product for 3 weeks at −60 °C. mp: 98.85 °C; 1 H NMR (500.1 MHz, CDCl 3 , 296 K): δ 7.68-7-72 (m, 2 H, Ph- H ), 7.40-7.44 (m, 3 H, Ph- H ), 6.97 (s, 2 H, Mes- H ), 6,94 (s, 2 H, Mes- H ), 2.54 (s, 6 H, o -C H 3 ), 2.35 (s, 3 H, p -C H 3 ), 2.34 (s, 3 H, p -C H 3 ), 2.09 (s, 6 H, o -C H 3 ); 13 C{ 1 H} NMR (125.7 MHz, CDCl 3 , 296 K): δ 171 (s, C q), 167.49 (s, C q), 145.35 (s, C q), 140.75 (s, C q), 136.31 (s, C q), 133.61 (s, C q), 133.34 (s, C q), 132.39 (s, C q), 131.07 (s, C H-Ph), 130.12 (s, C H-Ph), 128.86 (s, C H-Ph), 128.52 (s, C q), 128.10 (s, C H-Mes), 127.71 (s, C H-Mes), 23.55 (s, p - C H 3 -Mes), 21.6 (s, o - C H 3 -Mes), 21.28 (s, o - C H 3 -Mes), 20.6 (s, p - C H 3 -Mes); 11 B{ 1 H} NMR (160.4 MHz, CDCl 3 , 296 K): δ 32.8 (s). IR (hexane solution): 1,708 cm −1 (B–C–C ring-breathing—calculated to be at 1,759 cm −1 via DFT methods); analysis (calcd, found for C 26 H 27 B): C (89.15, 88.76) H (7.77, 7.69). Preparation of platinum-borirene adduct 2 In a Schlenk flask 100 mg (0.149 mmol) tetrakis(triethylphosphine)platinum(0) and 52.4 mg (0.149 mmol) borirene 1 were heated under vacuum (1×10 −3 mbar) to 60°C for 6 h. The solids were dissolved in 2 ml tetrahydrofuran (THF). After removing all volatiles the residue was extracted with hexane (2×2 ml) and filtered. The solution was stored at −30 °C for 35 days. The platinum–borirene adduct was isolated as a pale yellow solid (70 mg, 0.089 mmol, 63%). Crystals suitable for X-ray analysis were obtained after storing a hexane solution of the product for 3 days at −30°C. mp: 151°C; 1 H NMR (500.1 MHz, C 6 D 6 , 296 K): δ 7.51–7.50 (m, 2 H, m - H -Ph), 7.07–7.04 (m, 2 H, o - H -Ph), 6.95-6.93 (m, 1 H, p - H -Ph), 6.85 (s, 2 H, o - H -MesB), 6.82 (s, 2 H, o - H -MesC), 2.59 (s, 6 H, m -C H 3 -MesB), 2.25 (s, 3 H, p -C H 3 -MesB), 2.19 (s, 3 H, p -C H 3 -MesC), 2.15 (s, 6 H, m -C H 3 -MesC), 1.48-1.41 (m, 6 H, P2C H 2 ), 1.30-1.27 (m, 6 H, P1C H 2 ), 0.93 (dt, 9 H, 1 J H-H =7.28, 3 J P-H =15.0, P2CH 2 C H 3 ), 0.90 (dt, 9 H, 1 J H-H =7.28, 3 J P-H =15.0, P1CH 2 C H 3 ); 13 C{ 1 H} NMR (125.7 MHz, C 6 D 6 , 296 K): δ 189.29 (br s, Cq vin -B), 166.21 (br s, Cq vin -Pt), 147.18 (s, C q-Ph), 142.64 (br s, C q-MesB), 140.48 (br s, C q-MesC), 138.23 (s, o - C q-MesB), 135.13 (s, p - C q-MesB), 134.13 (s, p - C q-MesC), 132.32 (s, o - C q-MesC), 128.58 (s, m - C H-MesC), 127.68 (s, o - C H-Ph), 127.64 (s, m - C H-MesB), 126.27 (s, p - C H-Ph), 23.07 (s, o - C H 3 -Mes), 21.26 (s, p - C H 3 -Mes), 21.08 (s, p - C H 3 -Mes), 20.43 (s, o - C H 3 -Mes), 19.66–19.33 (m, P C H 2 ), 8.98-8.71 (m, PCH 2 C H 3 ), the assignment of the carbon nuclei in the 13 C{ 1 H} NMR spectrum was aided by two-dimensional 1 H- 13 C correlation spectra; 11 B{ 1 H} NMR (160.4 MHz, C 6 D 6 , 296 K): δ 39.62 (s); 31 P{ 1 H} NMR (202.4 MHz, C 6 D 6 , 296 K): δ 14.46 (s, 1 J Pt-P =2112 Hz), 10.73 (s, 1 J Pt-P =3188 Hz); 195 Pt{ 1 H} NMR (107.0 MHz, C 6 D 6 , 296 K): δ −4763.94 (dd, 1 J Pt-P1 =3188 Hz, 1 J Pt-P2 =2112 Hz); IR (hexane solution): 1531 cm −1 (C=C stretch, calculated to be at 1583 cm −1 ); analysis (calcd., found for C 38 H 57 BP 2 Pt): C (58.39, 58.38), H (7.35, 7.40). Reaction of 2 with diphenylacetylene A mixture of 2 (11.3 mg, 0.0145 mmol) and 2 eq. diphenylacetylene (10 mg, 0.029 mmol) was dissolved in C 6 D 6 (0.4 ml). NMR spectroscopy showed immediate and quantitative conversion to free borirene 1 and [Pt(PhC 2 Ph)(PEt 3 ) 2 ] [57] . 31 P{ 1 H} NMR (81.01 MHz, C 6 D 6 , 296 K): δ 11.97 (s, 1 J Pt-P =1650.8 Hz). Crystallographic details The crystal data of 1 ( Supplementary Data 1 ) and 2 ( Supplementary Data 2 ) were collected on a Bruker Apex diffractometer with a CCD area detector and graphite monochromated Mo Kα radiation. The structure was solved using direct methods, refined with the Shelx software package [58] and expanded using Fourier techniques. All non-hydrogen atoms were refined anisotropically. Hydrogen atoms were assigned to idealized positions and were included in structure factor calculations. Electrochemical details All cyclic voltammetry experiments were conducted in an argon-filled glovebox, using a Gamry Instruments Reference 600 potentiostat. A standard three-electrode cell configuration was employed using a platinum disk working electrode, a platinum wire counter electrode, and a silver wire, separated by a Vycor tip, serving as the reference electrode. Formal redox potentials are reported versus the ferrocene/ferrocenium (Fc 0/+ ) redox couple obtained by using decamethylferrocene (Me 10 Fc) as an internal standard and accounting for the difference in formal redox potentials in the respective solvent media ( E 1/2 = E 1/2 (Fc 0/+ ) E 1/2 (Me 10 Fc 0/+ )=+455 mV in THF with 0.1 M n Bu 4 NPF 6 as the supporting electrolyte). [59] Compensation for resistive losses ( iR drop) was employed for all measurements. Platinum complex 2 was studied by cyclic voltammetry in THF with n Bu 4 NPF 6 as the supporting electrolyte. Complex 2 exhibits an irreversible oxidation at 0.03 V versus ferrocene/ferrocenium (Fc/Fc + ) assigned to the Pt(0)/Pt(II) redox couple and 2 corresponding cathodic waves of small magnitude at −0.67 V and −1.28 V ( Supplementary Fig. S4 ). The observed oxidation potential compares well with data for other bis(phosphine) platinum(0) systems, supporting the Pt(0) oxidation state assignment in complex 2 . Oxidation potentials vs Fc 0/+ of relevant compounds are as follows: [(Ph 3 P) 2 Pt(C 2 H 4 )] ( E pa =0.07 V), [Pt{P(CH 2 Cy) 3 } 2 ] ( E pa =−0.03 V), [Pt(PCy 3 ) 2 ] ( E pa =−0.04 V) and trans -[PtCl 2 {P(CH 2 Cy) 3 } 2 ] ( E pc =−3.0 V). How to cite this article: Braunschweig, H. et al . Unsupported boron–carbon σ-coordination to platinum as an isolable snapshot of σ-bond activation. Nat. Commun. 3:872 doi: 10.1038/ncomms1884 (2012).